Pharmacological modulation of the AKT/microRNA-199a-5p/CAV1 pathway ameliorates cystic fibrosis lung hyper-inflammation In cystic fibrosis (CF) patients, hyper-inflammation is a key factor in lung destruction and disease morbidity. We have previously demonstrated that macrophages drive the lung hyper-inflammatory response to LPS in CF mice, because of reduced levels of the scaffold protein CAV1 with subsequent uncontrolled TLR4 signalling. Here we show that reduced CAV1 and, consequently, increased TLR4 signalling, in human and murine CF macrophages and murine CF lungs, is caused by high microRNA-199a-5p levels, which are PI3K/AKT-dependent. Downregulation of microRNA-199a-5p or increased AKT signalling restores CAV1 expression and reduces hyper-inflammation in CF macrophages. Importantly, the FDA-approved drug celecoxib re-establishes the AKT/miR-199a-5p/CAV1 axis in CF macrophages, and ameliorates lung hyper-inflammation in Cftr -deficient mice. Thus, we identify the AKT/miR-199a-5p/CAV1 pathway as a regulator of innate immunity, which is dysfunctional in CF macrophages contributing to lung hyper-inflammation. In addition, we found that this pathway can be targeted by celecoxib. Lung hyper-inflammation, characterized by increased production of interleukin (IL)-8, IL-6 and other pro-inflammatory cytokines, decreased anti-inflammatory cytokines and a greater number of immune cells [1] , is recognized as a key factor in cystic fibrosis (CF) lung destruction. Therefore, several anti-inflammatory drugs have been tested in CF patients. Among these, high-dose treatment with the non-steroidal anti-inflammatory drug (NSAID) ibuprofen is, to date, the only drug proven to be effective in slowing the progression of lung disease [2] , and increasing life expectancy in CF patients [3] . Unfortunately, the high doses needed for achieving a beneficial outcome are associated with several side effects, limiting its use among CF patients. In the last few years, tremendous progress has been made in identifying small molecules (potentiators) that effectively increase the activity of the defective cystic fibrosis transmembrane conductance regulator (CFTR) channel, the protein affected in CF, which has resulted in therapy for a small number of CF patients. In addition, other small molecules effective in improving the plasma membrane localization (correctors) of the most common CFTR mutant (F508del) are currently in clinical trials. Nevertheless, it is not yet clear whether CFTR corrector and potentiator therapies will suppress inflammation in CF [4] . Thus, there is a need to identify new therapeutic interventions for controlling hyper-inflammation in CF. Although it is thought that hyper-inflammation in CF is a consequence of chronic infection, growing evidence suggests that CFTR, in addition to its very well-established role in ion transport, also regulates signalling in receptors involved in the immune response [5] , [6] , [7] . CFTR also modulates signalling in MΦs [8] , which are central mediators of the inflammatory response, contributing both to initiation and resolution of inflammation. Indeed, we and others have demonstrated that CF MΦs contribute directly to the increased production of pro-inflammatory cytokines in mouse lungs, and that expression of wild-type (WT) CFTR in MΦs is sufficient to ameliorate the exaggerated lung inflammation in CF mice [9] , [10] . We were the first group to report that CFTR modulates the trafficking and signalling of the innate immune receptor Toll-like receptor 4 (TLR4) in MΦs. We found that in the absence of CFTR, TLR4 signalling is increased leading to an enhanced pro-inflammatory response [7] . More recently, these findings were corroborated in CF airway epithelial cells, suggesting that CFTR controls TLR4 signalling in several cell types [11] . Subsequently, we determined that murine and human CF MΦs, mucosal MΦs from human CF nasal polyp biopsies and lung tissues from knockout (KO) and F508del/F508del mice fail to induce expression of the scaffold protein caveolin 1 (CAV1) in response to lipopolysaccharides (LPSs) [12] . Due to reduced CAV1, haeme-oxygenase 1 (HO-1), a key stress response protein involved in balancing cellular redox status and inflammation, does not translocate to the plasma membrane, where it normally acts to downregulate TLR4 signalling [12] , [13] . Thus, the CAV1/HO-1 protective pathway is altered in CF cells and, by preventing downregulation of TLR4 signalling, this defect contributes to the perpetuation of the vicious cycle of hyper-inflammation and oxidative stress in CF [12] . The mechanism/s by which dysfunctional CFTR alters CAV1 induction in response to inflammatory triggers remains to be elucidated. MicroRNAs (miRNAs) are small noncoding RNAs that exert post-transcriptional gene regulation activity by targeting messenger RNAs. MiRNAs are involved in various fundamental biological processes and deregulation of miRNAs results in pathological conditions. Importantly, miRNAs play a central role in the regulation of innate host defence and the inflammatory response [14] and their disregulation contributes to chronic inflammatory lung diseases, including asthma, chronic obstructive pulmonary disease (COPD), idiopathic pulmonary fibrosis, CF and bronchiectasis, which are all characterized by an abnormal innate host defence response to environmental stimuli and infection [15] . Several miRNAs are abnormally expressed in CF-affected primary airway epithelial cells. These miRNAs fall into two main categories: miRNAs that modulate levels of functional CFTR directly (for example, miRs 145, 223, 494, 509, 101) or indirectly (for example, miR138), and several others that affect the innate immune response by altering downstream signalling of TLRs (for example, miRs 126, 93, 155) or by weakening humoral defence (miR-31; summarized in refs 16 , 17 , 18 , 19 ). We hypothesized that reduced CAV1 induction in CF MΦs, which affects TLR4 signalling, could be due to altered miRNA-dependent post-transcriptional regulation. Among miRNAs that are predicted to target the 3′-untranslated region (UTR) of CAV1 and that are conserved among species, microRNA 199a-5p (miR-199a-5p) has been validated for its ability to target CAV1 (ref. 20 ). Based on this evidence, we studied miR-199a-5p expression in CF. Here, we demonstrate, using a combination of pharmacological and genetic tools that lack CFTR in MΦs is associated with high levels of miR-199a-5p due to blunted phosphatidylinositol 3-kinase (PI3K)/protein kinase B (AKT) signalling in response to TLR4 activation. Increased levels of miR-199a-5p, targeting the 3′-UTR of CAV1, interfere with induction of CAV1 in response to inflammatory triggers, ultimately leading to ineffective negative feedback of TLR4 signalling and hyper-inflammation. Thus, we have identified a novel dysregulated signalling pathway in CF that contributes to lung hyper-inflammation. Importantly, we show that celecoxib (Celebrex), an Food and Drug Administration (FDA)-approved NSAID used in the treatment of osteoarthritis and rheumatoid arthritis and not yet tested for efficacy in CF patients or in other chronic inflammatory lung diseases, restores the AKT/miR-199a-5p/CAV1 pathway in CF MΦs and ameliorates lung hyper-inflammation in Cftr -deficient mice. Given the leading role of TLR4 signalling in MΦs to control lung innate host defence, dysfunctions in the AKT/miR-199a-5p/CAV1 pathway in MΦs may play a role in the pathobiology of several chronic inflammatory lung diseases. Increased levels of miR-199a-5p in CF MΦs and lung tissues We have previously shown that CF MΦs treated with LPS have increased TLR4 signalling because of reduced CAV1 expression [12] . The mechanism/s by which lack of functional CFTR in MΦs interferes with CAV1 induction in response to inflammatory triggers remained to be investigated. In lung fibroblasts [20] and myoblasts [21] , miRNA-199a-5p was recently identified as a potent regulator of CAV1 expression by specifically binding its 3′-UTR. Thus, we tested whether increased levels of miR-199a-5p are responsible for reduced CAV1 in bone marrow-derived (BMD) MΦs isolated from Cftr -deficient mice (referred to hereafter as CF MΦs), and whether miR-199a-5p plays a role in regulating TLR4 signalling. We observed that LPS exposure decreased miR-199a-5p by 50% in WT murine MΦs after 2 h, and this effect persisted for 4 h ( Fig. 1a ). In contrast, in CF MΦs, the LPS-induced downregulation of miR-199a-5p was completely abrogated, and CF MΦs had a modest, but statistically significant, increase in miR-199a-5p ( Fig. 1a ). In contrast, miR-802, another miRNA with a predicted recognition site for CAV1, was not affected by LPS stimulation and no differences were observed between WT and CF MΦs ( Supplementary Fig. 1a ). Importantly, expression of the hypoxia-inducible factor 1alpha (Hif-1α), which is a known target of miR-199a-5p in lung tissues [22] and myocytes [23] , was decreased twofold in CF MΦs exposed to LPS compared with WT cells ( Supplementary Fig. 1b ), indicating that miR-199a-5p is differentially upregulated. 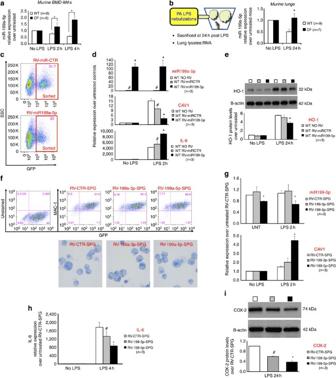Figure 1: miR-199a-5p, an upstream regulator of CAV1 and TLR4 signalling, is increased in CF. (a) MiR-199a-5p relative expression (quantitative PCR (qPCR)) in murine WT (white bars) and CF (black bars) BM-derived MΦs, untreated or treated with LPS. (b) Cartoon representation of thein vivotreatment and qPCR for miR-199a-5p in lung lysates from WT and CF-KO mice untreated or treated with LPS. (c) Flow cytometry dot-plots of WT murine MΦs infected with RV-miR-GFP (miR-CTR) vector control (top) or RV-miR-199a-5p-GFP (bottom), showing FACS sorting scheme. (d) qPCR for miR-199a-5p (top), CAV1 (middle) and IL-6 (bottom) in RVs infected and sorted WT MΦs, untreated or treated with LPS; data are compared with uninfected WT MΦs. (e) Western blot (WB) and densitometric analysis for HO-1 in uninfected or RVs infected WT MΦs, untreated or treated with LPS. (f) Flow cytometry dot-plots of CF murine MΦs infected with RV-sponge (SPG)-control, RV-199a-3p-SPG or RV-199a-5p-SPG, showing puromycin-selected GFP- positive population expressing the MΦs marker MAC-1 (top panel) and MΦs cytospun cells stained with Giemsa, demonstrating the absence of morphological abnormalities among different MΦ populations (bottom panel). qPCR for miR-199a-5p and for CAV1 (g) and IL-6 (h) in RV-SPG-infected and puromycin-selected CF MΦs, untreated or treated with LPS. (i) WB and densitometric analysis for COX-2 in RV-SPG-infected and puromycin-selected CF MΦs, untreated or treated with LPS. For qPCR, miR-199a levels are normalized to RNU6B and CAV1/IL-6 expression to S18. For WB, protein fold increase is normalized to β-actin. Unless indicated differently, for each experiment, the data are the result of three experimental biological repeats or are representative of three experimental biological repeats. Statistical analyses were conducted using one-sided two-samplet-tests. Error bars indicate standard deviation. Symbols * and ♯ indicate a statistically significant difference among the experimental group and control group with aPvalue <0.05. Figure 1: miR-199a-5p, an upstream regulator of CAV1 and TLR4 signalling, is increased in CF. ( a ) MiR-199a-5p relative expression (quantitative PCR (qPCR)) in murine WT (white bars) and CF (black bars) BM-derived MΦs, untreated or treated with LPS. ( b ) Cartoon representation of the in vivo treatment and qPCR for miR-199a-5p in lung lysates from WT and CF-KO mice untreated or treated with LPS. ( c ) Flow cytometry dot-plots of WT murine MΦs infected with RV-miR-GFP (miR-CTR) vector control (top) or RV-miR-199a-5p-GFP (bottom), showing FACS sorting scheme. ( d ) qPCR for miR-199a-5p (top), CAV1 (middle) and IL-6 (bottom) in RVs infected and sorted WT MΦs, untreated or treated with LPS; data are compared with uninfected WT MΦs. ( e ) Western blot (WB) and densitometric analysis for HO-1 in uninfected or RVs infected WT MΦs, untreated or treated with LPS. ( f ) Flow cytometry dot-plots of CF murine MΦs infected with RV-sponge (SPG)-control, RV-199a-3p-SPG or RV-199a-5p-SPG, showing puromycin-selected GFP- positive population expressing the MΦs marker MAC-1 (top panel) and MΦs cytospun cells stained with Giemsa, demonstrating the absence of morphological abnormalities among different MΦ populations (bottom panel). qPCR for miR-199a-5p and for CAV1 ( g ) and IL-6 ( h ) in RV-SPG-infected and puromycin-selected CF MΦs, untreated or treated with LPS. ( i ) WB and densitometric analysis for COX-2 in RV-SPG-infected and puromycin-selected CF MΦs, untreated or treated with LPS. For qPCR, miR-199a levels are normalized to RNU6B and CAV1/IL-6 expression to S18. For WB, protein fold increase is normalized to β-actin. Unless indicated differently, for each experiment, the data are the result of three experimental biological repeats or are representative of three experimental biological repeats. Statistical analyses were conducted using one-sided two-sample t -tests. Error bars indicate standard deviation. Symbols * and ♯ indicate a statistically significant difference among the experimental group and control group with a P value <0.05. Full size image MiR-199a-5p/CAV1 levels were also modulated by the TLR5 ligand flagellin, which together with LPS plays a major role in driving inflammation in CF. As observed for LPS, CF MΦs exposed to flagellin have reduced CAV1 expression and increased levels of miR-199a-5p, suggesting that the miR-199a-5p/CAV1 pathway is downstream of the MyD88-dependent innate immune response ( Supplementary Fig. 1c ). MiR-199a-5p has recently been linked to α1-antitrypsin deficiency and to the unfolded protein response (UPR) [24] . At the experimental conditions used and at the time points assessed, we did not observe statistically significant differences between WT and CF MΦs in the induction of the UPR regulator gene Grp78 or of the signal transducer ATF6 ( Supplementary Fig. 1d ). This does not exclude that miR-199a-5p may affect the levels of UPR-associated transcriptome after prolonged exposure to LPS or in the presence of the F508del protein. The miR-199a-5p and miR-199a-3p mature miRNA sequences arise from a common stem loop structure that is highly conserved across vertebrate species. Although to a lesser extent than miR-199a-5p, miR199a-3p, which arises from the 3′ arm of the miR199a hairpin and does not have the predicted consensus sequences for the CAV1 3′-UTR [21] , was also modulated by LPS and increased levels were observed in CF MΦs compared with controls ( Supplementary Fig. 1e , left panel). MiR-199b-5p, another miRNA with similar sequence homology to miR-199a-5p but transcribed from a different genetic locus [21] , was expressed at very low levels compared with miR-199a-5p in MΦs. LPS induced a modest and transient increase in miR-199b-5p but no differences were observed between WT and CF cells ( Supplementary Fig. 1e , right panel). We then assessed the transcriptional levels of the stem-loop miR-199a precursors. Expression of both the a-1 and a-2 precursors was modulated by LPS. MiR-199a-2 stem loop precursors had a pattern of expression comparable to that observed for miR-199a-5p, with decreased levels in response to LPS in WT MΦs. Furthermore, miR-199a-2 downregulation was absent in CF MΦs ( Supplementary Fig. 1f ). Thus, the variation in mature miR-199a-5p levels between WT and CF MΦs in response to LPS may be predominantly due to differential expression of the miR-199a-2 stem-loop precursor sequence. 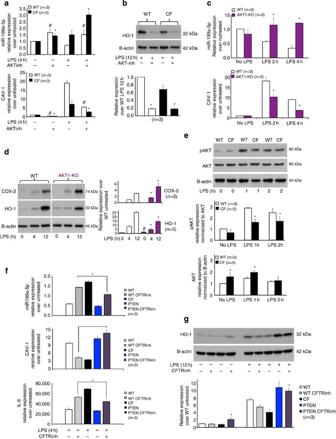Figure 2: Induction of the PI3K/AKT signalling in CF MΦs rescues the miR-199a-5p/CAV1 axis and reduces hyper-inflammation. (a) Quantitative PCR (qPCR) for miR-199a-5p (top panel) and CAV1 (bottom panel) or (b) WB and densitometric analysis for HO-1 in WT and CF-KO murine MΦs untreated or treated with LPS, in the absence or presence of the PI3K/AKT inhibitor LY294002. (c) qPCR for miR-199a-5p (top panel) and CAV1 (bottom panel) or (d) WB and densitometric analysis for COX-2 and HO-1 in WT and AKT1-KO murine MΦs untreated or treated with LPS. (e) WB and densitometric analysis for phospho-AKT and total AKT in WT and CF-KO murine MΦs untreated or treated with LPS. (f) qPCR for miR-199a-5p (top panel), CAV1 (middle panel) and IL-6 (bottom panel) or WB and densitometric analysis for HO-1 (g) in WT, WT+CFTR inhibitor CFTRinh172, CF-KO, PTEN-KO and PTEN-KO+ CFTRinh172 MΦs untreated or treated with LPS. Symbols * indicate a statistically significant difference among WT+CFTRinh172 and PTEN-KO+ CFTRinh172 MΦ groups. For qPCR, miR199a levels are normalized to RNU6B and CAV1 and IL-6 expression to S18. For WB, protein fold increase is normalized to β-actin or AKT (pAKT). Unless indicated differently, for each experiment, the data are the result of three experimental biological repeats or are representative of three experimental biological repeats. Statistical analyses were conducted using one-sided two-samplet-tests. Error bars indicate standard deviation. Symbols * and ♯ indicate a statistically significant difference among the experimental group and control group withPvalues <0.05. Figure 2: Induction of the PI3K/AKT signalling in CF MΦs rescues the miR-199a-5p/CAV1 axis and reduces hyper-inflammation. ( a ) Quantitative PCR (qPCR) for miR-199a-5p (top panel) and CAV1 (bottom panel) or ( b ) WB and densitometric analysis for HO-1 in WT and CF-KO murine MΦs untreated or treated with LPS, in the absence or presence of the PI3K/AKT inhibitor LY294002. ( c ) qPCR for miR-199a-5p (top panel) and CAV1 (bottom panel) or ( d ) WB and densitometric analysis for COX-2 and HO-1 in WT and AKT1-KO murine MΦs untreated or treated with LPS. ( e ) WB and densitometric analysis for phospho-AKT and total AKT in WT and CF-KO murine MΦs untreated or treated with LPS. ( f ) qPCR for miR-199a-5p (top panel), CAV1 (middle panel) and IL-6 (bottom panel) or WB and densitometric analysis for HO-1 ( g ) in WT, WT+CFTR inhibitor CFTR inh 172, CF-KO, PTEN-KO and PTEN-KO+ CFTR inh 172 MΦs untreated or treated with LPS. Symbols * indicate a statistically significant difference among WT+CFTR inh 172 and PTEN-KO+ CFTR inh 172 MΦ groups. For qPCR, miR199a levels are normalized to RNU6B and CAV1 and IL-6 expression to S18. For WB, protein fold increase is normalized to β-actin or AKT (pAKT). Unless indicated differently, for each experiment, the data are the result of three experimental biological repeats or are representative of three experimental biological repeats. Statistical analyses were conducted using one-sided two-sample t -tests. Error bars indicate standard deviation. Symbols * and ♯ indicate a statistically significant difference among the experimental group and control group with P values <0.05. Full size image We next tested the expression of miR-199a-5p in the lungs of CF mice in response to inhaled LPS, which we have already reported have reduced CAV-1 expression [9] , [12] (see also Fig. 3h ). Consistent with the in vitro results, we found that LPS challenge caused miR-199a-5p downregulation, which was not observed in CF lung tissues ( Fig. 1b ). A similar pattern of expression was observed for miR-199a-3p, whereas miR-802 levels, although increased by LPS, were not different between WT and CF mice ( Supplementary Fig. 1g ). Taken together, these results suggest that miR-199a is dysregulated in CF MΦs and in CF murine lungs, and that elevated levels of miR-199a may play an important role in CF-related lung hyper-inflammation. 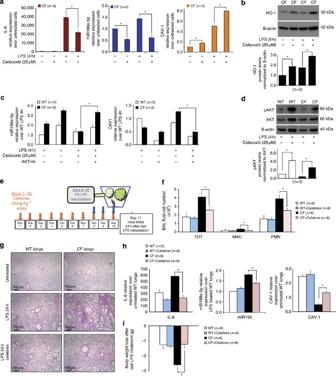Figure 3: Celecoxib rescues the miR-199a-5p/CAV1 pathways by stimulating PI3K/AKT signalling in CF MΦs, and decreases the lung hyper-inflammatory response to LPS in CF-affected mice. (a) Quantitative PCR (qPCR) for IL-6 (left), miR-199a-5p (middle) and CAV1 (right) and (b) WB and densitometric analysis for HO-1 in CF murine MΦs untreated or treated with LPS, in the absence or presence of celecoxib. (c) qPCR for miR-199a-5p (left) and CAV1 (right) in WT and CF murine MΦs treated with LPS, in the presence or absence of celecoxib and of PI3K/AKT inhibitor LY294002. (d) WB and densitometric analysis for AKT, pAKT and β-actin in WT and CF murine MΦs treated with LPS for 4 h in the presence or absence of celecoxib. (e)In vivoexperiment schematic representation; total and differential BAL fluid cell number (f), haematoxylin/eosin staining in paraffin-embedded lung tissues (g), qPCR for IL-6, miR-199a-5p and CAV1 (h) and body weight loss (i) from WT and CF mice treated chronically (10 days) with celecoxib (Celebrex) and then challenged with LPS for 3 days. Mice were killed 24 h after last nebulization. For qPCR, miR-199a levels are normalized to RNU6B and CAV1 and IL-6 expression to S18. For WB, protein fold increase is normalized to β-actin or total AKT (pAKT). For thein vitroexperiments, the data are the result of three experimental biological repeats; for thein vivostudy, three mice were used for each group, and the experiment was repeated independently twice (total: six mice per group). Statistical analyses were conducted using one-sided two-samplet-tests (qPCR) or two-sample unequal variancet-tests (BAL fluid cell numbers). Error bars indicate standard deviation. The symbol * indicates a statistically significant difference among groups withPvalues <0.05. Images were acquired using an Olympus BX51 microscope with a × 4 objective; scale bar is 100 μm. Figure 3: Celecoxib rescues the miR-199a-5p/CAV1 pathways by stimulating PI3K/AKT signalling in CF MΦs, and decreases the lung hyper-inflammatory response to LPS in CF-affected mice. ( a ) Quantitative PCR (qPCR) for IL-6 (left), miR-199a-5p (middle) and CAV1 (right) and ( b ) WB and densitometric analysis for HO-1 in CF murine MΦs untreated or treated with LPS, in the absence or presence of celecoxib. ( c ) qPCR for miR-199a-5p (left) and CAV1 (right) in WT and CF murine MΦs treated with LPS, in the presence or absence of celecoxib and of PI3K/AKT inhibitor LY294002. ( d ) WB and densitometric analysis for AKT, pAKT and β-actin in WT and CF murine MΦs treated with LPS for 4 h in the presence or absence of celecoxib. ( e ) In vivo experiment schematic representation; total and differential BAL fluid cell number ( f ), haematoxylin/eosin staining in paraffin-embedded lung tissues ( g ), qPCR for IL-6, miR-199a-5p and CAV1 ( h ) and body weight loss ( i ) from WT and CF mice treated chronically (10 days) with celecoxib (Celebrex) and then challenged with LPS for 3 days. Mice were killed 24 h after last nebulization. For qPCR, miR-199a levels are normalized to RNU6B and CAV1 and IL-6 expression to S18. For WB, protein fold increase is normalized to β-actin or total AKT (pAKT). For the in vitro experiments, the data are the result of three experimental biological repeats; for the in vivo study, three mice were used for each group, and the experiment was repeated independently twice (total: six mice per group). Statistical analyses were conducted using one-sided two-sample t -tests (qPCR) or two-sample unequal variance t -tests (BAL fluid cell numbers). Error bars indicate standard deviation. The symbol * indicates a statistically significant difference among groups with P values <0.05. Images were acquired using an Olympus BX51 microscope with a × 4 objective; scale bar is 100 μm. Full size image MiR-199a-5p regulates CAV1 levels and TLR4 signalling in MΦs To prove that miR-199a-5p regulates CAV1 expression in LPS-stimulated MΦs, and modulates the inflammatory response, we overexpressed miR-199a-5p in WT cells. Murine WT BMD-progenitor cells were infected with the retrovirus vector (RV) pMSCV-miR-199a5p-PGK-EGFP (RV-miR-199a-5p) or pMSCV-PGK-EGFP control (RV-miR-CTR) and differentiated in MΦ colony-stimulating factor. Overexpression of miR-199a-5p had no effect on MΦ differentiation, as demonstrated by the unchanged MAC-1 expression between infected (green fluorescent protein (GFP)-positive) and uninfected (GFP-negative) cells ( Supplementary Fig. 1h ). GFP-positive cells were sorted ( Fig. 1c ), plated and treated with LPS for 2 h. RV-miR-199a-5p-infected cells highly upregulated miR-199a-5p in both untreated and LPS-treated conditions with a very slight increase in miR-199a-5p levels in RV-miR-CTR-infected cells ( Fig. 1d , upper panel). Although LPS treatment upregulated CAV1 expression 15-fold in controls, overexpression of miR-199a-5p resulted in a dramatic decrease in CAV1 expression in response to LPS. A small decrease of CAV1 expression was also observed in RV-miR-CTR-infected cells ( Fig. 1d , middle panel). Consistent with our previous findings, decreased CAV1 expression was associated with a hyper-inflammatory response to LPS, as shown by increased IL-6 ( Fig. 1d , lower panel) and decreased amounts of the downstream target HO-1 ( Fig. 1e ). Next, we tested whether knocking down miR-199a-5p would abrogate the hyper-inflammatory response in CF MΦs. We used RV vectors that expressed RNA containing complementary binding sites for miR-199a-5p (miRNA sponge). The miR-199a-5p sponge (RV-miR-199a-5p-SPG) should specifically bind and competitively inhibit miR-199a-5p binding to mRNA targets, thus providing stable and specific miR-199a-5p inhibition [25] . As a control, we used a RV-control-sponge (RV-CTR-SPG), which does not target miRNAs, or a RV-miR199a-3p-sponge (RV-miR-199a-3p-SPG), which specifically inhibits miR-199a-3p but not miR-199a-5p. These vectors also encode enhanced green fluorescent protein (EGFP) and puromycin-resistance genes, allowing for selection of infected MΦs. Up to 89% of the cells were positive for GFP and for the MΦ markers MAC-1 ( Fig. 1f , upper panel) or F4/80 ( Supplementary Fig. 1i ), and no alterations of MΦ morphology were observed after infection ( Fig. 1f , lower panel). The sequestration of miRNAs by sponges can trigger their degradation [25] . Accordingly, the miR-199a-5p sponge caused a 30% decrease of miR-199a-5p expression in primary transduced CF MΦs in the presence or absence of LPS, but had no effect on miR-199a-3p ( Fig. 1g , upper panel). Similarly, miR-199-3p sponge decreased miR-199a-3p levels, but had no effect on miR-199a-5p ( Supplementary Fig. 1j ). CF MΦ transduction with miR-199a-5p sponge (but not with miR-199a-3p sponge) led to a 2.2-fold increase in CAV1 expression in response to LPS compared with control vectors ( Fig. 1g , lower panel). Consistent with induction of CAV1 expression, sequestration of miR-199a-5p in CF-MΦs reduced TLR4 signalling, as demonstrated by 2.5-fold decreased IL-6 expression ( Fig. 1h ) and 2.5-fold decreased COX-2 protein ( Fig. 1i ). Interestingly, downregulation of miR-199a-3p has some anti-inflammatory effects, which are CAV1-independent ( Fig. 1g–i ). In summary, elevated miR-199a-5p level in WT MΦs is sufficient to abrogate CAV1 expression in response to LPS and to promote the hyper-inflammatory response, whereas downregulation of miR-199a-5p in CF MΦs re-establishes CAV1 expression and reduces the pro-inflammatory response. AKT signalling is required for miR-199a-5p/CAV1 modulation Next, we investigated the signalling pathway required for miR-199a-5p downregulation in response to LPS. In cardiac myocytes, downregulation of miR-199a-5p in response to oxygen-related stressors is dependent on PI3K/protein kinase B (AKT; PI3K/AKT) pathway activation [26] . In addition, increased levels of miR-199a-5p and decreased pAKT were observed in lung tissue samples of patients with COPD [22] . In MΦs, the PI3K/AKT pathway is induced by LPS and its activation regulates different immune functions [27] . Among these, PI3K/AKT negatively regulates TLR4 signalling [28] , [29] . Thus, we investigated whether the downregulation of miR-199a-5p in WT MΦs in response to LPS was dependent on PI3K/AKT pathway activation and whether this pathway was altered in CF MΦs. WT and CF MΦs treated with the PI3K inhibitor (LY294002) had increased miR-199a-5p ( Fig. 2a , upper panel), and reduced CAV1 ( Fig. 2a ; lower panel), both at steady-state and in response to LPS. HO-1 induction in response to LPS was affected by LY294002 treatment as well, whereas its very low expression at steady-state was not altered ( Fig. 2b and Supplementary Fig. 2a ). LY294002 also increased miR-199a-3p levels in response to LPS ( Supplementary Fig. 2b ), suggesting that the PI3K/AKT regulates miR-199a at the expression level. In mammals, the AKT family consists of three isoforms, AKT1/PKBα, AKT2/PKBβ and AKT3/PKBγ. We chose to test the AKT1 isoform since this isoform is involved in regulation of LPS tolerance in MΦs via miRNAs [30] . We show that MΦs differentiated from the BM of homozygous AKT1-KO mice have increased levels of miR-199a-5p and decreased CAV1 expression in response to LPS compared with WT cells ( Fig. 2c ). Consistent with defective TLR4-negative feedback, AKT1-KO MΦs have increased IL-6 ( Supplementary Fig. 2c ) and COX-2 expression ( Fig. 2d ) in response to LPS. HO-1 protein level was elevated in untreated AKT1-KO MΦs, but its induction in response to LPS was blunted compared with WT cells ( Fig. 2d ). Together, these data suggest that negative regulation of TLR4 signalling via miR199-5p/CAV1 is, at least in part, PI3K/AKT1 dependent. These results led us to assess AKT phosphorylation in CF MΦs challenged with LPS. We found that CF MΦs, although they expressed abundant total AKT, had a modest but statistically significant reduction of AKT phosphorylation at serine 473 compared with WT MΦs after 1 and 2 h. In addition, this difference persisted at 4 h of LPS challenge ( Fig. 3d ). Thus, blunted PI3K/AKT signalling in response to LPS observed in CF MΦs may contribute to defective regulation of the miR199-5p/CAV1 axis and hyper-inflammation. To test the direct effect of AKT phosphorylation on miR-199a levels, CF MΦs were treated with increasing doses of the AKT agonist SC79 for 4 h. SC79 decreased miR-199a-5p levels in a dose-dependent manner, which correlated with augmented AKT signalling. High doses of SC79 also had effects on miR-199-3p, but not on miR-802 ( Supplementary Fig. 2d ). Next, we tested whether rescuing PI3K/AKT signalling in CF environment would restore a controlled inflammatory response. To this end, we used BMD-MΦs from phosphatase and tensin homologue (PTEN)-KO mice, which have constitutive upregulation of phosphoAKT and are hypo-responsive to signals associated with MΦ activation [31] . PTEN KO MΦs ( Fig. 2f , blue bars) have slightly lower miR-199a-5p levels and slightly higher CAV1 expression than WT cells in response to LPS ( Fig. 2f , white bars). Both WT cells treated with the CFTR inhibitor CFTR inh 172 (ref. 32 ; Fig. 2f , grey bars) and CF cells ( Fig. 2f , black bars) had high miR-199a-5p and reduced CAV1 expression compared with WT controls. Therefore, chemical inhibition of CFTR in WT cells recapitulates the CF phenotype, as we have also demonstrated previously [7] . Importantly, CFTR inhibition in a PTEN-KO background ( Fig. 2f , violet bars) caused reduction of miR-199a-5p and increased in CAV1 expression compared with WT MΦs treated with CFTR inh 172 ( Fig. 2f , grey bars). In addition, CFTR inhibition in PTEN-KO MΦs also decreased LPS-induced inflammation, as shown by lowered IL-6 expression ( Fig. 2f , bottom panel), and increased HO-1 protein production ( Fig. 2g ), in a PI3K/AKT-dependent manner ( Supplementary Fig. 2e ). These data suggest that stimulation of the PI3K/AKT signalling pathway in CF MΦs rescues the hyper-inflammatory response to LPS. Celecoxib targets the AKT/miR-199a-5p/CAV1 pathway Celecoxib (Celebrex), an FDA-approved selective COX-2 inhibitor used in the treatment of osteoarthritis, rheumatoid arthritis and pain management, has been reported to activate PI3K/AKT and mitochondrial redox signalling to enhance HO-1-mediated anti-inflammatory activity in vascular endothelium [33] . Celecoxib also induces CAV1 expression [34] , potentially in a COX-2 inhibition-independent manner [35] . Thus, we tested the hypothesis that celecoxib could decrease TLR4 signalling in CF MΦs via modulation of the miR-199-5p/CAV1 axis. CF MΦs were pretreated overnight with celecoxib before LPS treatment. In addition to the expected downregulation of the pro-inflammatory response, as shown by reduced IL-6 expression ( Fig. 3a , left panel, dark red bars), celecoxib-treated CF MΦs had a statistically significant decrease in miR-199a-5p expression ( Fig. 3a , middle panel, blue bars), as well as increased CAV1 mRNA ( Fig. 3a , right panel, orange bars) and HO-1 protein production ( Fig. 3b ) compared with vehicle-treated (dimethylsulphoxide (DMSO)) CF cells. The highest induction of the HO-1 pathway without cell toxicity was observed at a dose of 25 μM ( Supplementary Fig. 2f ). The ability of celecoxib to downregulate miR-199a-5p and increase CAV1 was prevented by pre-treatment of CF MΦs with the PI3K/AKT inhibitor LY294002 ( Fig. 3c ), and activation of the PI3K/AKT pathway was increased in celecoxib pre-treated CF MΦs challenged with LPS ( Fig. 3d ). Therefore, celecoxib modulates the miR-199a-5p/CAV1 signalling pathway in CF MΦs challenged with LPS in a PI3K/AKT-dependent manner. Unlike celecoxib, at 25 μM, the classic NSAID ibuprofen fails to efficiently rescue the miR-199a/CAV1 pathway in CF MΦs treated with LPS. Modulation of miR-199a/CAV1 was observed at a higher ibuprofen dosage (100 μM), which, however, had more broad and nonspecific effects, as it also affected miR-802 expression ( Supplementary Fig. 2g ). Ibuprofen was also less efficient at inducing HO-1 compared with celecoxib ( Supplementary Fig. 2h ). Because celecoxib abrogated the hyper-inflammatory response of CF MΦs to LPS, we next tested its effect on LPS-induced hyper-inflammation in CF murine lungs [7] , [9] . Mice were treated orally with the FDA-approved drug celecoxib (Celebrex) for 10 days (25 mg kg −1 per day) or with vehicle (apple juice) alone ( Supplementary Table 1 ). At this dosage, Celebrex has anti-inflammatory effects in rat lungs with smoke-induced emphysema [36] . Mice received nebulized LPS, as previously described [9] , from days 8 to 10 and killed 24 h after the last nebulization (day 11; Fig. 3e ). CF mice treated with celecoxib had reduced inflammatory responses to LPS compared with vehicle-treated CF mice, as demonstrated by reduced total broncho-alveolar lavage (BAL) fluid cell number, macrophages (MAC) and neutrophils (PMN; Fig. 3f ). In addition, histological analysis of lung tissues stained with haematoxylin and eosin confirmed decreased inflammation in mice treated with celecoxib ( Fig. 3g ). Decreased inflammatory BAL cells were associated with reduced IL-6 expression in celecoxib-treated CF lung tissues ( Fig. 3h , left panel). Importantly, celecoxib treatment in LPS-challenged CF mice reduced miR-199a-5p ( Fig. 3h , middle panel), and increased CAV1 expression ( Fig. 3h , right panel) in lung tissues compared with vehicle-treated CF tissues. Pre-treatment with celecoxib also reduced weight loss associated with LPS challenge in CF mice ( Fig. 3i ). Celecoxib had minimal effects on WT mice ( Fig. 3g–i ). In contrast to celecoxib, ibuprofen treatment (50 mg kg −1 for 10 days), despite some effects on the inflammatory response to LPS compared with vehicle-treated CF animals, was not effective in modulating the miR-199a-5p/CAV1 pathway or in preventing LPS-induced weight loss in CF mice ( Supplementary Fig. 3c,d and Supplementary Table 1 ). Finally, to test whether celecoxib’s protective action to LPS is due, at least in part, to the AKT-dependent downregulation of the miR-199a-5p in vivo , AKT1-KO mice ( Supplementary Table 1 ) were treated with celecoxib or vehicle alone and then challenged with LPS, as described in Fig. 4e . As previously reported [37] , AKT1-KO mice had robust lung neutrophilic inflammation in response to LPS ( Supplementary Fig. 3b ). Upregulation of miR-199a-5p and downregulation of CAV1 were even more pronounced than what was observed in CF mice, as was LPS-induced weight loss. Celecoxib treatment in AKT1-KO mice had a modest effect in reducing BAL cell number and IL-6 expression, but no restoration of the miR-199a-5p/CAV1 pathway and no protection against weight loss were observed ( Supplementary Fig. 3a–d ). Thus, celecoxib-dependent protection against weight loss and lung hyper-inflammation in response to LPS requires activation of the AKT/miR-199a-5p/CAV1 pathway. 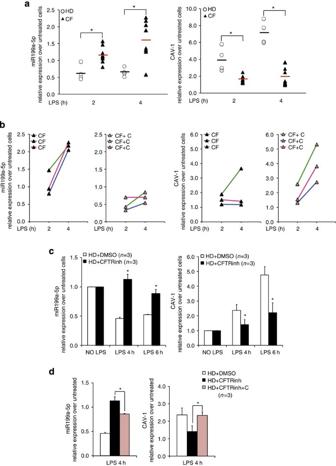Figure 4: miR-199a-5p/CAV1 axis is defective in human CF MΦs and can be modulated by celecoxib pre-treatment. (a) Quantitative PCR (qPCR) for miR-199a-5p (left) and CAV1 (right) in PB-derived MΦs isolated from four healthy donors (HDs each donor sample is indicated with a white dot) and eight CF patients (each patient sample is indicated with a black triangle), untreated or treated with LPS for 2 and 4 h. Relative expression is calculated over untreated controls and the average relative expression is indicated by a black (HD) or a red (CF) bar. (b) qPCR for miR-199a-5p and CAV1 in human CF MΦs (CF hMΦs) treated with LPS without (left panels) or with celecoxib (25 μM) pretreatment (right panels; indicated as CF+C); each colour represents a distinct CF patient. (c) qPCR for miR-199a-5p (left) and CAV1 (right) in human MΦs differentiated from non-CF CD34-positive mobilized PB cells and conditioned with the CFTR inhibitor CFTRinh172 (HD+CFTRinh) or with vehicle alone (HD+DMSO). (d) qPCR for miR-199a-5p (left) and CAV1(right) in HD+DMSO and HD+CFTRinhpretreated with celecoxib (25 μM; HD+CFTRinh+C). The miR-199a-5p levels are normalized to RNU6B and CAV1 expression to S18. For the experiments with CD34-positive mobilized PB cells the data are the result of three experimental biological repeats. Statistical analyses were conducted using one-sided two-samplet-tests. Error bars indicate standard deviation. The symbol * indicates a statistically significant difference among groups withPvalues <0.05. Figure 4: miR-199a-5p/CAV1 axis is defective in human CF MΦs and can be modulated by celecoxib pre-treatment. ( a ) Quantitative PCR (qPCR) for miR-199a-5p (left) and CAV1 (right) in PB-derived MΦs isolated from four healthy donors (HDs each donor sample is indicated with a white dot) and eight CF patients (each patient sample is indicated with a black triangle), untreated or treated with LPS for 2 and 4 h. Relative expression is calculated over untreated controls and the average relative expression is indicated by a black (HD) or a red (CF) bar. ( b ) qPCR for miR-199a-5p and CAV1 in human CF MΦs (CF hMΦs) treated with LPS without (left panels) or with celecoxib (25 μM) pretreatment (right panels; indicated as CF+C); each colour represents a distinct CF patient. ( c ) qPCR for miR-199a-5p (left) and CAV1 (right) in human MΦs differentiated from non-CF CD34-positive mobilized PB cells and conditioned with the CFTR inhibitor CFTR inh 172 (HD+CFTR inh ) or with vehicle alone (HD+DMSO). ( d ) qPCR for miR-199a-5p (left) and CAV1(right) in HD+DMSO and HD+CFTR inh pretreated with celecoxib (25 μM; HD+CFTR inh +C). The miR-199a-5p levels are normalized to RNU6B and CAV1 expression to S18. For the experiments with CD34-positive mobilized PB cells the data are the result of three experimental biological repeats. Statistical analyses were conducted using one-sided two-sample t -tests. Error bars indicate standard deviation. The symbol * indicates a statistically significant difference among groups with P values <0.05. Full size image Celecoxib modulates miR-199a-5p in human CF MΦs We then tested whether miR-199a-5p levels are also elevated in human MΦs isolated from CF patients. We isolated peripheral blood (PB)-derived MΦs from eight CF donors ( Supplementary Table 2 ) and from four healthy donor (HD) controls. Cells were treated with LPS for 2 and 4 h. The fold change in expression of miR-199a-5p and CAV1 in response to LPS for each individual’s MΦs was compared with its own untreated control. Despite variability in response to LPS across individuals, we found that miR-199a-5p levels were elevated, and CAV1 expression was decreased in MΦs from CF individuals when compared with HD MΦs, as we have observed in murine cells ( Fig. 4a ). Pre-treatment of CF MΦs with celecoxib (colour lines indicate three different donors) decreased miR-199a-5p levels, and increased CAV1 expression ( Fig. 4b ). To investigate whether the inability of CF MΦs to upregulate CAV1 in response to LPS is a consequence of nonfunctional CFTR, we treated human MΦs differentiated from CD34-positive mobilized PB cells with CFTR inh 172 or with vehicle (DMSO) alone. Non-CF human MΦs treated with CFTR inh 172 phenocopied CF MΦs, with increased miR-199a-5p, decreased CAV1 induction ( Fig. 4c ) and increased IL-6 expression ( Supplementary Fig. 3e ) in response to LPS. Thus, in human MΦs, the hyper-inflammatory dysfunction is directly linked to the presence of functional CFTR. Furthermore, overnight pre-treatment with celecoxib decreased miR-199a-5p, and increased CAV1 expression in non-CF human MΦs treated with CFTR inh 172 ( Fig. 4d ). In summary, we have validated that the miR-199a-5p/CAV1 axis is defective in primary human diseased CF MΦs and that celecoxib treatment can rescue this defect. Hyper-inflammation is recognized as a critical factor in lung tissue deterioration, and lung function decline in CF patients, which contributes to morbidity and mortality [1] . Although CF mice do not fully recapitulate human CF lung disease, they are a very good model for studying CF-related GI manifestations, ion transport defects and systemic inflammation [38] . In fact, CF mice manifest hyper-inflammation in the lungs [9] , [39] , pancreas [40] and intestine [41] at baseline, or after exposure to various inflammatory triggers. Thus, CF mouse models recapitulate aspects found in human CF hyper-inflammation. The CFTR gene is expressed in secretory epithelia of the body and, at lower levels, in other cell. CFTR protein is detected in murine [9] , [42] and human [43] , [44] MΦs and CFTR-like Cl − conductance has been recorded in monocytes/MΦs [7] , [42] , [43] , suggesting that in these cells CFTR functions as a cAMP-dependent chloride channel. Several studies have shown that CF MΦs contribute directly to lung hyper-inflammation [9] , [10] . CFTR MΦs also display defective bacterial killing [42] , [44] , [45] due to dysfunctional autophagy [46] . Thus, CF MΦs exhibit several cell-autonomous immune dysfunctions that contribute to CF lung disease, which make MΦs potential targets for effective CF treatments. We have shown that hyper-secretion of pro-inflammatory cytokines in CF MΦs is due to reduced levels of the scaffold protein caveolin 1 (CAV1) that causes TLR4 signalling upregulation [7] , [12] . CAV1 is a multi-functional structural protein involved in the formation of specialized plasma membrane lipid rafts [47] , in mediating clathrin-independent endocytosis and cholesterol trafficking, and in mediating bacterial and viral immunity [48] , [49] . CAV1 also binds to and controls the location, and activity of several signalling molecules, including TNFR1, ERK1/2, Src, nitric oxide synthase and glucocorticoid receptors [50] . Importantly, CAV1 binds to, and negatively regulates TLR4 in MΦs [13] , and this protective mechanism is defective in CF MΦ [12] . CAV1 also downregulates transforming growth factor (TGF)-β signalling [51] , a key pathway with relevance to lung fibrosis. Consistent with the observed interdependency between decreased CAV1 and TGF-β-driven lung fibrosis, increased TGF-β signalling has recently been found in the lungs of CF patients [52] . Here we show that miR-199a-5p, an upstream direct regulator of CAV1, is increased in CF MΦ and CF murine lungs exposed to inflammatory triggers. MiR-199a-5p modulates several signalling pathways such as TGF-β [20] and WNT [21] and elevated levels of miR-199a-5p have been linked to alteration of various cellular processes, such as suppressed autophagy [53] , increased apoptosis [54] and defective hypoxic response [23] , most of which are also dysregulated in CF [55] , [56] . Here, for the first time, we link miR-199a-5p levels with TLR4 signal regulation in MΦs showing that elevated levels of miR-199a-5p, by impairing CAV1-dependent TLR4 signalling suppression, contribute to CF-related lung hyper-inflammation ( Fig. 1 ). Furthermore, using genetic and biochemical techniques, we demonstrated that the miR-199a-5p/CAV1 axis in MΦs and mouse lung tissue is modulated by PI3K/AKT signalling and that in CF MΦs, the blunted AKT phosphorylation in response to LPS contributes to cellular accumulation of miR-199a-5p and decreased CAV1. Thus, the miR-199a-5p/CAV1 axis participates in the hyper-inflammatory response to LPS ( Fig. 2 and Supplementary Figs 2 and 3 ). This is an intriguing observation, since TLR4 activation in MΦs induces the binding between MyD88 and the PI3K regulatory subunit, which ultimately activates AKT signalling. The PI3K/AKT signalling pathway plays a critical role in feedback inhibition of TLR4 signalling [28] , [30] , and dysfunctional PI3K/AKT activation in response to LPS is sufficient to enhance the mitogen-activated protein kinase pathway and nuclear factor-κB nuclear translocation [28] , [29] , which we previously reported is enhanced in LPS-treated CF MΦs [7] . Thus, although uncontrolled AKT signalling can lead to a variety of cancers, induction of this pathway in response of inflammatory stressors is fundamental for balancing immune cell functions. Importantly, genetic restoration of the AKT signalling in a CF background is sufficient for decreasing the hyper-inflammatory response to LPS ( Fig. 2 ). Treatment of alveolar MΦs isolated from CF patients with the insulin-like growth factor 1, a potent AKT activator, enhances their capability to kill bacteria [57] . Thus, blunted AKT signalling may also play a role in the defective bactericidal activity of CF MΦs. This pathway may also be defective in CF airway epithelial cells as a recent study demonstrated that pharmacological or genetic inhibition of CFTR in airway epithelial cells prevents PI3K plasma membrane localization [58] , which is necessary for AKT phosphorylation. Our data in genetic mouse models suggest that, among the different AKT isoforms, AKT1 signalling is involved in regulating miR-199-5p/CAV1 and TLR4 signalling, which is consistent with its leading role in orchestrating neutrophil recruitment in mice [37] and in modulating the abundance of several miRNAs that regulate TLR4 signalling (for example, miR-155, let7e and miR-125b) [30] . Our data provide evidence that the FDA-approved NSAID celecoxib (Celebrex), which is currently not considered for treatment in CF or other chronic lung inflammatory diseases, stimulates the AKT/miR-199a-5p/CAV1 signalling pathway, decreasing lung hyper-inflammation and preventing the excessive weight loss associated with LPS exposure in Cftr -deficient mice ( Fig. 3 ). The fact that this drug has favourable effects in Cftr -null mice suggests that celecoxib’s mechanism/s of action circumvents the need for functional CFTR. Thus, this drug may have a broad therapeutic application, which may include benefits for CF patients with nonsense mutations. Importantly, at the doses used, celecoxib had minimal effects in modulating lung inflammation in WT mice ( Fig. 3 ), suggesting a CF environment-dependent mode of action. Our data show that celecoxib’s beneficial effects are, at least in part, due to modulation of the AKT/miR-199a-5p/CAV1 pathway, in addition to COX-2 inhibition. Also, genetic downregulation of miR-199a-5p in CF MΦs decreased COX-2 protein levels ( Fig. 1 ), suggesting that celecoxib regulates not only COX-2 enzymatic function, but also its expression. Highlighting the relevance of this observation, Cftr -null mice have inherently higher levels of COX-2 (ref. 59 ). Celecoxib is an intriguing small molecule also because it appears to bind to the hydrophobic acyl core of phospholipid membranes, changing physical properties of membranes and potentially modifying the activity of membrane-bound proteins [60] , [61] , which may explain in part celecoxib’s effect on TLR4 signalling. However, further studies are necessary to better understand the COX-2-independent mechanisms of celecoxib. Celecoxib is more efficient than ibuprofen in modulating the miR199-5p/CAV1 pathway, in reducing lung hyper-inflammation and in preventing LPS-induced weight loss in CF mice ( Supplementary Fig. 3c,d ). In CF patients, ibuprofen has been proven to be efficient in preserving lung function and weight loss, but this is achieved with high doses that maintain the drug plasma concentration at 50–100 μg ml −2 . We do not know whether in our mouse study the ibuprofen plasma concentration was maintained substantially overtime. Our in vivo studies support the hypothesis that AKT1 is required for miR-199a-5p downregulation in response to LPS and that the celecoxib-dependent protection of weight loss and, partially, of hyper-inflammation in response to LPS, requires activation of this pathway. In CF patients, maintenance of body weight is critical for lung function preservation [62] , and impaired AKT signalling may contribute to the low body mass index in patients with CF, which may not only be caused by the loss of exocrine pancreatic function or by gut malabsorption [63] . In addition, AKT is a key metabolic modulator and defective AKT signalling is associated with insulin resistance [64] . Thus, this finding may be also relevant in the context of CF-related diabetes. In conclusion, our data provide mechanism-based evidence that celecoxib is a potential candidate for controlling lung hyper-inflammation in CF. Although Celebrex has a warning of increased risk of myocardial infarction, these adverse cardiovascular events appear similar among users of celecoxib and other classical NSAIDs [65] . In a large randomized clinical trial centred at the Cleveland Clinic, celecoxib is currently being compared with naproxen and ibuprofen for its overall benefit versus risk profile for treating osteoarthritis and rheumatoid arthritis (NCT00346216). In the context of chronic inflammatory lung diseases, elevated levels of miR-199a-5p or reduced expression of CAV1 has been reported in lung fibroblasts and monocytes of idiopathic pulmonary fibrosis [20] , scleroderma [66] and asthma [67] patients, and in lung endothelial cells of COPD patients [22] . Based on the evidence that components of the AKT/miR-199a-5p/CAV1 pathway are defective in several chronic inflammatory lung diseases, and given the leading role of MΦs’ TLR4 signalling to innate host defence response to environmental stimuli and infection, this study provides novel insights into the development and treatment of these inflammatory-based lung diseases. This study may be of particular relevance for COPD. In fact, cigarette smoke, the major cause of COPD, leads to systemic CFTR dysfunction [68] . In conclusion, we have identified the AKT/miR-199a-5p/CAV1 axis as an important regulatory pathway in MΦs that serves as a cellular protective mechanism and ensures immune-regulation in response to inflammatory triggers. Importantly, we demonstrate that this pathway is defective in CF, contributing to the hyper-inflammatory lung disease in Cftr -deficient mice. These dysfunctions in CF murine and human MΦs and in CF murine lungs are reversed by celecoxib treatment (summarized in Fig. 5 ). Our pre-clinical studies provide data suggesting that celecoxib would be beneficial for controlling lung disease in CF patients, thus supporting further testing in the clinical setting. 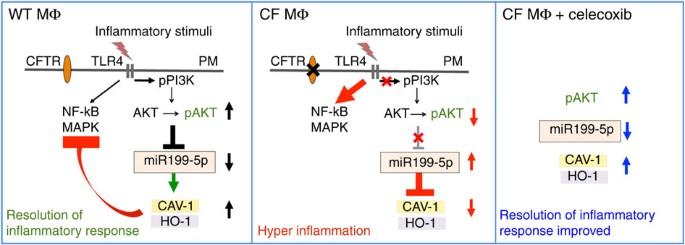Figure 5: TLR4 signalling negative feedback is regulated by the miR-199a-5p/CAV1 axis in an AKT-dependent manner and this pathway is altered in CF MΦs. TLR4 activation induces the PI3K/AKT pathway in MΦs, which downregulates microRNA miR-199a-5p, allowing expression of CAV-1 and subsequent negative feedback on the TLR4 pro-inflammatory cascade (nuclear factor-κB/mitogen-activated protein kinase signalling). In the absence of functional CFTR, MΦs have a blunted PI3K/pAKT signalling in response to TLR4 activation, which leads to accumulation of miR-199a-5p. Increased levels of miR-199a-5p, targeting the 3′-UTR of CAV1, interfere with induction of CAV1 in response to inflammatory triggers, ultimately leading to ineffective negative feedback of TLR4 signalling and hyper-inflammation. Celecoxib stimulates the AKT/miR-199a-5p/CAV1 pathway in CF murine and human MΦs, and decreases lung hyper-inflammation in Cftr-deficient mice. Figure 5: TLR4 signalling negative feedback is regulated by the miR-199a-5p/CAV1 axis in an AKT-dependent manner and this pathway is altered in CF MΦs. TLR4 activation induces the PI3K/AKT pathway in MΦs, which downregulates microRNA miR-199a-5p, allowing expression of CAV-1 and subsequent negative feedback on the TLR4 pro-inflammatory cascade (nuclear factor-κB/mitogen-activated protein kinase signalling). In the absence of functional CFTR, MΦs have a blunted PI3K/pAKT signalling in response to TLR4 activation, which leads to accumulation of miR-199a-5p. Increased levels of miR-199a-5p, targeting the 3′-UTR of CAV1, interfere with induction of CAV1 in response to inflammatory triggers, ultimately leading to ineffective negative feedback of TLR4 signalling and hyper-inflammation. Celecoxib stimulates the AKT/miR-199a-5p/CAV1 pathway in CF murine and human MΦs, and decreases lung hyper-inflammation in Cftr-deficient mice. Full size image Constructs The miR199a expression construct for miR-199a was cloned by PCR-amplification of genomic DNA with the following primers: 5′- CAGAACTTTCTCCAGATGCG -3′ and 5′- ATGGCAGACTGATAGGGCC -3′ PCR product was cloned into the pMIRWAY-puro and/or pMIRWAY-GFP vectors [69] (with MSCV LTR driving miRNA or sponge, and with PGK promoter driving puromycin resistance gene or GFP), through GateWay cloning (Invitrogen). The miRNA-inhibiting sponge sequences were obtained by oligonucleotide synthesis of five copies of either miR-199a-5p sites or miR-199a-3p sites, and cloned to generate sponges with ten copies of bulged binding sites. Specifically, the sequences were digested with either Sal I or Xho I and then ligated. Ten-copy sponge sequences were placed downstream of EGFP [25] and cloned into pMIRWAY-puro vector. Five-copy sponge oligo-sequences are listed below. miR-199a-5p: 5′- ATACAGATCTCCG TCGACGAACAGGTAGAAATAACACTGGGAAGAACAGATAGCAACAACACTGGGTTGAACAGGTAGGACTAACACT GGGACGAACAGATAGATACAACACTGGGCAGAACAGGTAGGAATAACACTGGGCTCGAGTAGG TGACACTATAGTTTCTCCAGATGCGAGCCGGGCGATCGCAGCACCATG -3′ miR-199a-3p: 5′- ATACAGATCTCCGTCG ACTAACCAATGAAATGACTACTGTAAAAAA CCAATCCTACCACTACTGCATTTAACCAATGGAGTG ACTACTGTGACAAACCAATCATAGCACTACTGCCACTA ACCAATGGTATGACTACTGTCTCGAGTAGGTGACACTA TAGGCAGCAAATGTGCCACGTCA GCGATCGCAGCACCATG -3′ Control vectors for miRNA are pMIRWAY-puro or pMIRWAY-GFP vectors without miRNA. Retroviral preparation and cell transduction Packing cells 293T (5 × 10 6 ) were transfected with plasmid mixture containing 10 μg of retroviral construct, 10 μg of gag/pol and 10 μg of VSVG constructs using FuGENE HD transfection reagent (Promega) following the instructions. Retrovirus was harvested in viral collection medium (DMEM with 10% heat-inactivated fetal bovine serum (FBS)+1% penicillin-streptomycin-glutamine+20 mM HEPES) for 3 days after transfection, twice a day. The viral collection medium was spun down at 1,500 r.p.m. for 5 min to remove 293T cells and concentrated with Amicon Ultra centrifugal filter-10 K (Millipore), at 4,000 r.p.m. for 2 h at 4 °C. Then, viral vectors were aliquoted and stored at −80 °C until use. Titre assessment Retrovirus titre was assessed using 293T cells. 1 × 10 6 cells were plated in 1.25 ml medium (DMEM supplemented with 10% heat-inactivated FBS; antibiotics and L -glutamine) together with 1 μl polybrene (10 mg ml −1 , American Bioanalytical) and with differing amounts of viral solution (none, 5, 15 and 30 μl). After spininfection (1,800 r.p.m. for 90 min), cells were cultured for 36–48 h before flow cytometry analysis for GFP-positive cells. The virus titre is calculated as follows: (GFP positive/100 × cell number)/Volume of virus (ml). For murine bone marrow cell transduction, we use a multiplicity of infection (MOI) virus/cells of 20:1. Briefly, 5 × 10 5 cells were cultured in six-well plates and exposed to each virus in 1 ml of serum-free medium. After spin infection (as above), cells were washed and incubated in serum-containing medium and in macrophage colony-stimulating factor (M-CSF) for 7 days. The GFP-positive cells were sorted (or selected with puromycin) and GFP-positive cells were then plated and subjected to treatments as indicated. Chemicals and reagents The following antibodies were used: rabbit anti-HO-1 (1:2,000 for western blot, Abcam); rabbit anti-COX-2 (1:1,000, Cell Signaling Technology); rabbit polyclonal anti-AKT and anti-pAKT (1:1,000, Cell Signaling Technology); rabbit anti-actin (1:5,000, Santa Cruz); anti-rabbit-HRP (1:2,000, Santa Cruz). Pseudomonas aeruginosa (PA) LPS (Sigma-Aldrich) was prepared in PBS at 100 × stock solution and used at a concentration of 100 ng ml −1 . Flagellin (Imgenex) was used at a concentration of 100 ng ml −1 ). CFTR inhibitor CFTR inh 172, a kind gift from Dr Alan Verkman) [32] , was freshly prepared in DMSO and used at concentration of 20 μM. The PI3K/AKT inhibitor LY294002 (Cell Signaling Technology) was prepared in DMSO and used at a concentration of 20 μM. The AKT Activator II, SC79 (Merck Millipore) was dissolved in DMSO and used at the final concentrations indicated. Celecoxib (Sigma-Aldrich) was dissolved in DMSO (stock solution 20 mM) and used at a final concentration of 25 μM. For the in vivo study, we used the FDA-approved branded celecoxib (Celebrex) at concentration of 25 mg kg −1 per mouse per day. Ibuprofen (Sigma-Aldrich) was dissolved in DMSO (stock solution 50 mM) and used at a final concentration of 25 or 100 μM. For the in vivo study, we used Walgreens Children's Ibuprofen Suspension (20 mg ml −1 ) at a final concentration of 50 mg kg −1 per mouse per day. Isolation and culture of MACs BMD murine MACs . BM collection was performed as described in ref. 9 . Briefly, BM cells were flushed with DMEM medium from the medullary cavities of the tibias and femurs using 25-G needle in sterile conditions. The BM suspension was filtered through a 70-μm cell strainer, and then mononuclear cells were enriched by the Ficoll-Paque method (Histopaque 1077 Sigma H8889). After overnight culture, the non-adherent cells were differentiated for 7 days in 20 ng ml −1 recombinant M-CSF (ConnStem Inc.). After 7 days, cells were detached and characterized by flow cytometry (F4-80 + /MAC-1 + population). The day before experiments, cells were plated according to the experimental design. Human MACs . Blood was obtained from HDs or from patients ( Supplementary Table 2 ) with CF during their annual check-up with informed consent in accordance with the Yale University Medical School Human Investigation Committee. MΦs were cultured as described in ref. 7 . Briefly, human mononuclear cells were isolated from whole blood by Ficoll-Paque method (Histopaque 1077 Sigma H8889), and seeded at 2 × 10 6 cells per well in 12-well plates in RPMI supplemented with 10% FBS and 40 ng ml −1 recombinant human M-CSF (ConnStem Inc.). Cells were fed every other day and split 1:1 every 4 days. After 1–2 weeks, cells were characterized by flow cytometry (CD14 + /CD45 + ) and morphology analyzed on cytospin. Before LPS treatment, cells were washed extensively with PBS, detached with Accutase (Innovative Cell Technology) and seeded at 0.5 × 10 6 cells per well across 12-well plates before LPS treatment. Human CD34 + cells were isolated by immunomagnetic selection (Miltenyi CliniMacs) from granulocyte colony-stimulating factor mobilized peripheral blood collected via apheresis with donor consent and differentiated into MΦs by 7 days of culture in human M-CSF (ConnStem Inc.). In the experiments in which we use CFTR inh 172 (20 μM) or celecoxib (25 μM), cells were pre-treated overnight with drugs or vehicle alone (DMSO) before adding LPS (100 ng ml −1 ). For inhibition of the PI3K/AKT pathway, cells were pre-treated with LY294002 (20 μM) or DMSO control for 1 h before LPS challenge. Mouse models All procedures were performed in compliance with relevant laws and institutional guidelines, and were approved by the Yale University Institutional Animal Care and Use Committee. Age and gender of all experimental mice are listed in Supplementary Table 1 . Transgenic CFTR −/− (B6.129P2-KOCftr tm1UNC ) mice were purchased from the Jackson Laboratory and bred in the Yale University Animal Facility. Mice are fully back-crossed to the C57BL/6 background. Littermate CFTR –/– mice were fed a liquid diet (Peptamen, Nestle) as previously described [9] . Non-CF littermate control mice used in the experiments were maintained on an identical diet to the CFTR −/− mice to eliminate nutritional status as a potential confounder ( Supplementary Table 1 ). The homozygous AKT1-KO mice are on a C57B/6 background; they were generated as previously described [70] , and provided by Dr Patty J. Lee. Mice (AKT1-KO and WT) used for the in vivo study are listed in Supplementary Table 1 . The PTEN-KO mice (B6.129S4-Pten tm1Hwu ), for obtaining deletion of PTEN in blood cells, mice were crossed with VAV-Cre mice (B6.Cg-Tg-Vav1-cre-A2Kio/J; early stage of haematopoiesis). Both transgenic mice were originally purchased from the Jackson Laboratory and provided by Dr Diane S. Krause. BM cells were isolated at 6–8 weeks of mouse age. In vivo experiment and BAL fluid collection and analysis For the in vivo study, WT, CF or AKT1-KO mice were treated orally with Celebrex, ibuprofen or with vehicle alone ( Supplementary Table 1 ). One capsule of Celebrex (100 mg) was dissolved in 14 ml of apple juice, and diluted in liquid food (Peptamen) at a dose of 25 mg kg −1 per mouse; ibuprofen suspension (20 mg ml −1 ) was diluted in Peptamen at a final concentration of 50 mg kg −1 per mouse per day. Food was changed daily for the time indicated ( Fig. 3e ). On day 8, WT, CF and AKT1-KO mice received LPS (Sigma L8643) over 3 days (a dose a day). LPS (12.5 mg) was administered with a nebulizer (Pulmo-Aide Compressor, Natallergy). Five millilitres of solution were nebulized over 15 min (ref. 9 ). During the 3 days of LPS nebulization, Celebrex was administered (25 mg kg −1 ) via oral gavage 4 h after each nebulization. At the times indicated, mice were killed. BAL fluid was collected using standard methods. The total and differential cell counts in the BAL of LPS-treated mice were assessed by counting, by morphological analysis on BAL cell cytospin preps and by flow cytometry analysis. After cardiac perfusion with PBS supplemented with heparin, the left lung lobes were inflated, harvested and paraffin embedded; the right lobes were snap frozen in liquid nitrogen and used for RNA/protein isolation. RT–PCR and expression analysis Cells were lysed in Triazol and total RNA was isolated from 1 × 10 6 cells using QiagenRNAMini Kits (Qiagen), following the instructions. Lung tissues were homogenized before RNA isolation. For cDNA analysis (Roche Molecular Biochemical), 2 μg total RNA was reverse-transcribed using iScript cDNA Synthesis Kit (Bio-Rad) following the manufacturer’s specifications. Real-time PCR analysis was performed with a Bio-Rad iCycler using TaqMan technology. Copy number was normalized by 18S and the relative expression to 0 (untreated cells) was calculated by ΔΔCt method. All TaqMan primers and probes were purchased from Applied Biosystem (Life Technology). For miRNA analysis, RNA was isolated from cells or tissues using the miRNeasy Mini Kit (Qiagen), and the reverse transcribed using the miSCript II RT kit (Qiagen). All miRNAs primers were purchased from Qiagen and quantitative PCR was performed using miScript SYBR green PCR kit (Qiagen). Copy number was normalized by RNU6B and the relative expression to untreated cells was calculated by ΔΔCt method. Unless indicated, the data are the result of at list three experimental biological repeats or are representative of three experimental biological repeats. Protein isolation and western blot Cold RIPA lysis buffer containing phosphatase inhibitors was added to cells. After 30 min of incubation in ice, the lysates were centrifuged and the supernatants recovered. An equal amount of protein was separated by electrophoresis on 10% Mini PROTEAN Gels (Bio-Rad), transferred to nitrocellulose membrane (Bio-Rad Laboratories) and hybridized using standard procedures. Horseradish Peroxidase-conjugated to IgG secondary antibodies (1:5,000, Santa Cruz) and Bio-Rad ECL was used for detection. The chemiluminescence imaging system ChemiDoc (Bio-Rad) and the Image lab software (Bio-Rad) were used for image acquisition and for signal quantification. Protein relative expression is normalized to β-actin or AKT (for pAKT). Images have been cropped for presentation. Full-size images are presented in Supplementary Fig. 4 . Statistical analysis Statistical analyses were conducted using one-sided two-sample t -tests or two-sample unequal variance t -tests ( in vivo studies). All experiments were performed in triplicate, unless indicated differently. Data are expressed as mean±standard deviation. A P value <0.05 was considered statistically significant. How to cite this article: Zhang, P.Z. et al . Pharmacological modulation of the AKT/microRNA-199a-5p/CAV1 pathway ameliorates cystic fibrosis lung hyper-inflammation. Nat. Commun. 6:6221 doi: 10.1038/ncomms7221 (2015).